Parallel T-cell cloning and deep sequencing of human MAIT cells reveal stable oligoclonal TCRβ repertoire Mucosal-associated invariant T (MAIT) cells are abundant in humans and recognize conserved bacterial antigens derived from riboflavin precursors, presented by the non-polymorphic MHC class I-like molecule MR1. Here we show that human MAIT cells are remarkably oligoclonal in both the blood and liver, display high inter-individual homology and exhibit a restricted length CDR3β domain of the TCRVβ chain. We extend this analysis to a second sub-population of MAIT cells expressing a semi-invariant TCR conserved between individuals. Similar to ‘conventional’ MAIT cells, these lymphocytes react to riboflavin-synthesizing microbes in an MR1-restricted manner and infiltrate solid tissues. Both MAIT cell types release Th0, Th1 and Th2 cytokines, and sCD40L in response to bacterial infection, show cytotoxic capacity against infected cells and promote killing of intracellular bacteria, thus suggesting important protective and immunoregulatory functions of these lymphocytes. Mucosal-associated invariant T (MAIT) cells represent up to 10% of circulating T cells in humans and are abundant in the gastrointestinal mucosa and liver [1] , [2] , [3] , [4] . Although MAIT cells are known to respond to Gram-positive bacteria, Gram-negative bacteria and yeasts [5] , [6] , and have antimicrobial potential [7] , [8] , [9] , [10] , there is no consensus on their physiological role. Antigen recognition by MAIT cells is mediated by an αβ T-cell receptor (TCR), in which the TCRVα chain comprises an almost-invariant Vα7.2-Jα33 ( TRAV1-2–TRAJ33 ) rearrangement paired with a limited number of TCRVβ chains [1] . These limited Vα-Vβ heterodimers are analogous to those of invariant natural killer T cells (iNKT) [11] , and the two cell populations also share expression of NK-related molecules such as CD161 in humans [2] , [12] and similarly acquire an effector/memory phenotype after birth [2] , [13] . In contrast to NKT cells, MAIT cells appear in the periphery following bacterial colonization [14] , suggesting that commensal bacteria-derived signals and/or antigens are important in sustaining their expansion and survival. MAIT cells recognize small microbial metabolites produced in the riboflavin pathway [15] , when presented as stimulatory complexes with the non-polymorphic major histocompatibility complex (MHC) class I-like related molecule 1 (MR1) [16] , [17] , [18] . Whether riboflavin-related metabolites are the only antigens stimulating MAIT cells, and how these antigens affect MAIT cell expansion and homeostasis remains to be elucidated. Another unresolved issue is how the TCR repertoire of the invariant T-cell populations is generated; whether it is predominantly antigen-driven or is dependent on random but convergent TCR gene rearrangement mechanisms. The almost-invariant TCRα chain of MAIT cells is evolutionarily conserved in mammals [14] , [19] and results from a single Vα-Jα rearrangement with a defined CDR3α length. In humans, some variation in the composition of the junction exists, suggesting a selective pressure operating at the protein level [14] . Nevertheless, a recent computer simulation of gene recombination events proposed that the invariant TCRα chains of MAIT and NKT cells can be generated by a recombination process involving various convergent mechanisms [20] . Studies comparing a limited number of TCR sequences have suggested that the TCRβ repertoire of MAIT cells might be biased toward Vβ2 ( TRBV20 ) and Vβ13 ( TRBV6 ), but failed to detect any preferential use of particular Jβ genes or identify the prevalence of defined CDR3β clonotypes [1] , [21] . However, the investigation of small numbers of MAIT TCR gene sequences precludes a thorough examination of the impact of antigen stimulation on shaping the TCR repertoire and of the TCRβ chain role in antigen recognition. MAIT cells are abundant in tissues exposed to microbial antigens, including the gut, liver and infected lung [2] , [5] , [22] . Their parallel abundance in the blood also suggests that they may recirculate between these organs. The oligoclonality of tissue-resident T lymphocytes was described long before the discovery of MAIT cells [23] , [24] , but it is unknown which of these oligoclonal T cells recognize microbial antigens presented by MR1. Here we define the TCRβ repertoire of MAIT cells in healthy humans by single cell cloning and mRNA deep sequencing experiments, and we show that a small number of clonotypes accounts for the majority of MAIT cells in both blood and liver. Furthermore, we describe a second population of MAIT cells expressing a different invariant TCRα chain. We also investigate the tissue distribution and effector functions of this novel subset in comparison with ‘conventional’ MAIT cells. Isolation and characterization of human MAIT cell clones Human MAIT cells are CD4-negative and express high levels of the NK-related marker CD161 (ref. 2 ). To establish MAIT cell clones, CD4 − CD161 high T cells were sorted from peripheral blood of a healthy donor (A) and cloned by limiting dilution. As iNKT and TCR γδ T cells also express CD161 and may lack CD4, they were excluded from sorting using antibodies specific for the TCR Vα24 (ref. 25 ) and Vδ2 chains [26] ( Supplementary Fig. 1a ). In preliminary experiments, a significant proportion of these CD4 − Vδ2 − Vα24 − CD161 + T cells upregulated surface expression of CD69 after co-culture with autologous monocytes infected with Escherichia coli ( Supplementary Fig. 1b ). When the individual T-cell clones were tested by PCR, 15 clones expressed the MAIT TCR Vα7.2-Jα33 rearrangement. Each T-cell clone was further characterized for the TCRVβ chain expressed and for surface expression of CD161, CD4 and CD8 by flow cytometry. Thirteen clones possessed Vβ2 ( BV2S1 according to ref. 27 or TRBV20-1 according to ref. 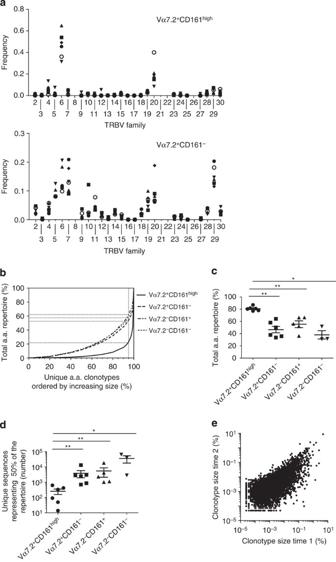Figure 1: MAIT cells are oligoclonal in human peripheral blood. (a) Vβ usage of sorted peripheral blood Vα7.2+CD161highMAIT cells (upper panel) and Vα7.2+CD161−control T cells (lower panel). IMGT nomenclature is used. Each point represents data from an individual healthy donor. (b) Distribution of clonotype sizes in Vα7.2+CD161highMAIT cells, and Vα7.2+CD161−, Vα7.2−CD161−and Vα7.2−CD161+control T cells from a representative donor. Data are plotted as percentage of total TCRβ amino acid (a.a.) repertoire versus the percentage of unique TCRβ amino-acid repertoire ordered by increasing size. They-value at which each curve intersects the dashed line (x=95%) represents the percent value of the total repertoire covered by 95% of unique clonotypes for each T-cell population. The graph shows that 5% of the most abundant clonotypes, evaluated as amino-acid, contribute 77% of the total TCRβ repertoire of Vα7.2+CD161highMAIT cells and only 38%, 56% and 52% of that of Vα7.2+CD161−, Vα7.2−CD161+and Va7.2−CD161−control T-cell populations, respectively. (c) Percentage of total TCRβ amino-acid repertoire represented by 5% of the largest unique amino-acid clonotypes for the indicated T-cell populations in all donors analysed. For every T-cell subset, each point represents a different donor. Bars indicate mean±s.e.m. (*P≤0.05, **P≤0.01, determined by Mann–WhitneyU-test). (d) Number of unique amino-acid sequences contributing the 50% of the total TCRβ amino-acid repertoire of the indicated T-cell populations. For every T-cell subset, each point represents data from a different donor. Bars indicate mean±s.e.m. (*P≤0.05, **P≤0.01, determined by Mann–WhitneyU-test). (e) Size of all individual TCRβ amino-acid clonotypes in Vα7.2+CD161highMAIT cells of a representative donor (3) analysed at two different time points with a 5-month interval. 28 ) or Vβ13 ( BV13S3 and BV13S5 or TRBV6-1 and TRBV6-4 ) chains, both reported to be preferentially expressed in MAIT cells [1] ( Table 1 ). Two clones instead expressed the Vβ7.2 ( BV7S2 or TRBV4-3 ) and Vβ16 ( BV16S1 or TRBV14 ) chains, respectively ( Table 1 ). The CD8 molecule was present in 13 clones, whereas one clone was CD4 − CD8 − ( Table 1 ). All T-cell clones were CD4 − and CD161 + ( Table 1 ), indicating that no bias was introduced by the sorting and cloning strategies. As MAIT cells recognize antigen-presenting cells (APC) infected with Gram-positive or Gram-negative bacteria [5] , [6] , three different bacterial strains were used to infect APC and study stimulation of the selected T-cell clones. Monocyte-derived dendritic cells or THP-1 myelomonocytic cells, which express surface MR1 ( Supplementary Fig. 1c ) were infected with E. coli (Gram-negative), Staphylococcus aureus (Gram-positive) and Mycobacterium smegmatis , and co-cultured with T-cell clones. Each tested clone responded to all the infected cells, regardless of APC type used and of the Vβ chain expressed by the clone ( Table 1 and Supplementary Fig. 1d ). Addition of anti-MR1 monoclonal antibodies (mAbs) inhibited T-cell responses ( Supplementary Fig. 1d ), but did not affect activation of MHC class II-restricted Mycobacterium tuberculosis -specific or CD1b-restricted M. tuberculosis -reactive T cells, used as controls ( Supplementary Fig. 1e ). Taken together, these data indicated that established Vα7.2-Jα33 T-cell clones are bona fide MAIT cells, as they express the prototypic markers of this population, their responses are restricted by MR1 and they recognize APC infected with riboflavin-producing bacteria. Table 1 Phenotype and amino acid TCR β sequences of V α 7.2-J α 33 T-cell clones from donor A. Full size table MAIT cells possess a limited TCRβ repertoire The analysis of TCRVβ sequences of 15 MAIT cell clones revealed that they represented only 7 different CDR3β amino acid clonotypes; moreover, three of these clonotypes together accounted for 11 clones (73%), being expressed in 5, 4 and 2 clones, respectively ( Table 1 ). As the T-cell clones were generated with neither previous stimulation nor in vitro expansion, it appeared that the circulating MAIT cell population might in fact originate from a small number of in vivo clonally expanded cells. To test this hypothesis, we investigated the TCRβ repertoire composition of the blood MAIT cells of healthy donors using RNA deep sequencing. MAIT lymphocytes were isolated by polychromatic flow cytometric cell sorting according to co-expression of TCRVα7.2 and CD161 high ( Supplementary Fig. 2 ), and TCRβ sequences were obtained from the sorted population. Non-MAIT cell subsets were defined by a combination of the same markers (Vα7.2 + CD161 − , Vα7.2 − CD161 + and Vα7.2 − CD161 − ) and were simultaneously sorted and analysed as controls ( Supplementary Fig. 2 ). These studies were performed in peripheral blood mononuclear cells (PBMC) from six healthy donors (1, 2B, 3, 4, 5 and 6) and in two samples of liver-associated mononuclear cells. The total sequences analysed were between 103,704 and 17,023,718 per donor and sorted T-cell population, and they showed a range of 2,258–438,029 unique sequences in all four T-cell subsets ( Supplementary Table 1 ). A strong bias in TCRVβ usage was observed in MAIT cells, as previously reported [1] . Vβ13 (TRBV6) and Vβ2 (TRBV20) families together accounted for 32–85% of the total MAIT cell repertoire, with some inter-donor variability ( Fig. 1a , upper panel). Heterogeneous Vβ usage was evident in Vα7.2 + CD161 − control T cells, thus excluding the possibility that the observed MAIT cell Vβ bias was associated with the presence of this TCRVα chain ( Fig. 1a , lower panel). Although a predominant expression of individual Jβ genes was not detected in MAIT cells compared with control T lymphocytes, significant differences were observed in the distribution of unique CDR3β amino acid clonotypes. In the MAIT cell population, 5% of the unique clonotypes with the largest size accounted for 77–82% of the total TCRβ repertoire ( Fig. 1b,c ). By contrast, the same 5% covered only 33–64%, 36–66% and 31–51% of the repertoire in Vα7.2 + CD161 − , Vα7.2 − CD161 + and Vα7.2 − CD161 − control T cells, respectively ( Fig. 1b,c ). These data indicated a marked oligoclonality of CDR3β amino acid clonotypes in MAIT cells, with relatively few clones accounting for the majority of the overall repertoire. Indeed, an average of 250 unique sequences were sufficient to represent 50% of the total MAIT cell repertoire, while 3,000–30,000 sequences on average covered the same proportion of the TCR repertoire in non-MAIT cell populations ( Fig. 1d ). Deep-sequence analysis performed on sorted Vα7.2 + CD161 high liver-associated MAIT lymphocytes, which can account for up to half the resident T-cell population of this organ [2] , [22] , revealed a distribution of CDR3β clonotypes comparable to that observed in peripheral blood ( Supplementary Fig. 3 ). In the two liver samples, 5% of the largest CDR3β clonotypes represented 84.3 and 81.6% of the total repertoire, respectively, thus suggesting that oligoclonality is a shared feature of both the liver-resident and circulating pool of MAIT cells. Figure 1: MAIT cells are oligoclonal in human peripheral blood. ( a ) Vβ usage of sorted peripheral blood Vα7.2 + CD161 high MAIT cells (upper panel) and Vα7.2 + CD161 − control T cells (lower panel). IMGT nomenclature is used. Each point represents data from an individual healthy donor. ( b ) Distribution of clonotype sizes in Vα7.2 + CD161 high MAIT cells, and Vα7.2 + CD161 − , Vα7.2 − CD161 − and Vα7.2 − CD161 + control T cells from a representative donor. Data are plotted as percentage of total TCRβ amino acid (a.a.) repertoire versus the percentage of unique TCRβ amino-acid repertoire ordered by increasing size. The y -value at which each curve intersects the dashed line ( x =95%) represents the percent value of the total repertoire covered by 95% of unique clonotypes for each T-cell population. The graph shows that 5% of the most abundant clonotypes, evaluated as amino-acid, contribute 77% of the total TCRβ repertoire of Vα7.2 + CD161 high MAIT cells and only 38%, 56% and 52% of that of Vα7.2 + CD161 − , Vα7.2 − CD161 + and Va7.2 − CD161 − control T-cell populations, respectively. ( c ) Percentage of total TCRβ amino-acid repertoire represented by 5% of the largest unique amino-acid clonotypes for the indicated T-cell populations in all donors analysed. For every T-cell subset, each point represents a different donor. Bars indicate mean±s.e.m. (* P ≤0.05, ** P ≤0.01, determined by Mann–Whitney U -test). ( d ) Number of unique amino-acid sequences contributing the 50% of the total TCRβ amino-acid repertoire of the indicated T-cell populations. For every T-cell subset, each point represents data from a different donor. Bars indicate mean±s.e.m. (* P ≤0.05, ** P ≤0.01, determined by Mann–Whitney U -test). ( e ) Size of all individual TCRβ amino-acid clonotypes in Vα7.2 + CD161 high MAIT cells of a representative donor (3) analysed at two different time points with a 5-month interval. Full size image To confirm the above observations, from the same Vα7.2 + CD161 high cells sorted from donor 2B and analysed in parallel for TCRβ gene deep sequencing, a second, independent, panel of MAIT cell clones was generated. 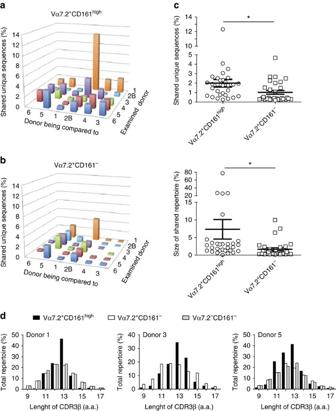Figure 2: MAIT cells exhibit a high degree of inter-individual TCRβ amino-acid sequence sharing and a bias in CDR3β length distribution. Percentage of unique amino-acid sequences shared between donor pairs in (a) Vα7.2+CD161highMAIT cells and (b) Vα7.2+CD161−control T cells. (c) Distribution of TCRβ repertoire overlapping between paired donors in Vα7.2+CD161highMAIT cells and Vα7.2+CD161−T cells in terms of unique amino-acid clonotypes (upper panel) and cumulative repertoire size (lower panel). Each point represents the percentage of unique amino-acid sequences (upper panel) and total TCRβ repertoire (lower panel) shared between two donors. Bars indicate mean±s.e.m. (*P≤0.05, determined by two-tailed unpaired Student’st-test with Welch’s correction). (d) Distribution of CDR3β lengths for the total TCRβ amino-acid (a.a.) repertoire (accounting for clonotype size) in the indicated sorted T-cell populations of three representative donors (1, 3 and 5). Within this panel, TCRβ sequence screening of 14 Vα7.2-Jα33-positive T-cell clones revealed only 8 different CDR3β clonotypes, 2 of which accounted for more than half of the cell clones ( Table 2 ). Deep sequencing showed that these eight sequences were highly frequent in the Vα7.2 + CD161 high cell subset from which the clones were derived, together representing >10% of the total TCRβ repertoire of MAIT cells from that donor, although being almost undetectable in the other control T-cell subsets ( Supplementary Table 2 ). Taken together, these findings provided a precise enumeration of the size of MAIT cell clonotypes in healthy donors and unequivocally demonstrated the oligoclonality of the MAIT population in the blood and liver. Table 2 Phenotype and amino acid TCR β sequences of V α 7.2-J α 33 T-cell clones from donor 2B. Full size table MAIT cell CDR3β clonotypes are stable in blood over time We next asked whether the oligoclonality observed in circulating MAIT cells is a stable or dynamic phenomenon. To address this issue, Vα7.2 + CD161 high cells were sorted from peripheral blood of three donors (3, 4 and 5) at two different time points separated by a 5-month interval, before parallel analysis of MAIT cell CDR3β clonotypes by mRNA deep sequencing ( Supplementary Table 1 ). In every individual, the observed CDR3β clonotypes were substantially unchanged, exhibiting comparable distribution and size within the total repertoire ( Fig. 1e and Supplementary Fig. 4 ). Importantly, the unique amino acid sequences common to the two time points represented between 99.6 and 99.9% of the total repertoire size. Few clonotypes were detected at one but not the other time point. These data suggested that within the investigated timeframe the majority of the circulating MAIT cell repertoire is stable in human peripheral blood. Inter-individual sharing of MAIT TCRβ clonotypes CDR3β clonotypes can be shared between different individuals [29] , implying a certain degree of TCR repertoire overlap in peripheral blood, although whether this similarly applies to the MAIT population is unknown. As MAIT cells uniquely recognize a common microbial antigen [15] and are oligoclonal, we hypothesized that they might also display a high degree of TCR repertoire overlap between different individuals. We therefore evaluated the extent of TCRβ repertoire sharing within the peripheral blood MAIT cell population between paired donors with respect to unique amino acid sequences and also to the cumulative repertoire size. In MAIT cells, 2±0.39% of the unique CDR3β amino acid clonotypes present in one individual were also present in a second individual ( Fig. 2a,c , upper panel). Furthermore, 7.3±2.7% of the total TCRβ repertoire overlapped in size between paired donors, with individuals sharing up to 80% ( Fig. 2c , lower panel). When the same analysis was performed in non-MAIT Vα7.2 + CD161 − and Vα7.2 − CD161 − cell populations, the proportion of unique CDR3β amino acid clonotypes and total size of shared TCRβ repertoire by paired donors dropped significantly to 1±0.19 and 0.65±0.29%, respectively, for unique clonotypes ( Fig. 2b,c , upper panel) and 1.6±0.4 and 0.52±0.12%, respectively, for repertoire size ( Fig. 2c , lower panel). Thus, the degree of TCRβ repertoire sharing between different individuals is substantially higher in MAIT than in non-MAIT cell populations. Figure 2: MAIT cells exhibit a high degree of inter-individual TCRβ amino-acid sequence sharing and a bias in CDR3β length distribution. Percentage of unique amino-acid sequences shared between donor pairs in ( a ) Vα7.2 + CD161 high MAIT cells and ( b ) Vα7.2 + CD161 − control T cells. ( c ) Distribution of TCRβ repertoire overlapping between paired donors in Vα7.2 + CD161 high MAIT cells and Vα7.2 + CD161 − T cells in terms of unique amino-acid clonotypes (upper panel) and cumulative repertoire size (lower panel). Each point represents the percentage of unique amino-acid sequences (upper panel) and total TCRβ repertoire (lower panel) shared between two donors. Bars indicate mean±s.e.m. (* P ≤0.05, determined by two-tailed unpaired Student’s t -test with Welch’s correction). ( d ) Distribution of CDR3β lengths for the total TCRβ amino-acid (a.a.) repertoire (accounting for clonotype size) in the indicated sorted T-cell populations of three representative donors (1, 3 and 5). Full size image We also evaluated the proportion of CDR3β clonotypes common to all the donors in MAIT and non-MAIT cell pools. Although in the latter group no public clonotypes were observed, in MAIT cells one identical CDR3β clonotype was detected in all analysed individuals, including the samples from the liver, further supporting the conclusion that some MAIT cell TCRβ sequences are commonly shared between different donors. CDR3β length distribution differs in MAIT and non-MAIT cells A recent study suggested that the TCRβ chain might be less important for MAIT cell stimulation than was previously thought [30] . To investigate whether the TCRVβ chains of MAIT cells have unique features, we compared the CDR3β length in MAIT and non-MAIT cells at amino acid level. In MAIT cells, a predominance of four CDR3β lengths was observed. In all donors, the dominant length was 13 amino acids, followed by 12, 11 and 14 with inter-individual heterogeneity ( Fig. 2d ). No significant bias was observed in control T-cell pools from the same individuals ( Fig. 2d ), indicating that the abundance of clonotypes with a restricted CDR3β length is a specific feature of MAIT lymphocytes. These observations were further supported by the analysis of the CDR3β amino acid clonotypes of all generated MAIT cell clones, which showed a size ranging between 11 and 14 amino acids, with only one exception ( Tables 1 and 2 ). The co-crystal of the TCR of MAIT cells and MR1 showed that CDR3β residues form van der Waals interactions with the MR1 α1 helix, thereby contributing to the overall interaction between the two proteins [31] , [32] . The preferential length of MAIT CDR3β sequences might contribute to optimal recognition of MR1–antigen complexes. Isolation of a second semi-invariant MAIT cell population From sorted Vα7.2 + CD161 high cells of donor 2B, we also isolated six T-cell clones, which were positively labelled by anti-Vα7.2 and anti-CD161 mAbs but did not express the Vα7.2-Jα33 transcript. 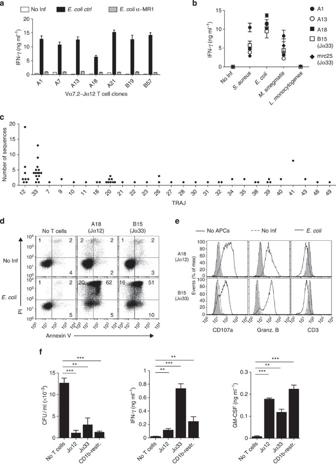Figure 3: Vα7.2-Jα12 T cells represent a subset of MAIT cells. (a) Seven Vα7.2-Jα12 T-cell clones were cultured with THP-1 cells that were either not infected (no Inf), or infected withE. coliin the presence of anti-MR1 (α-MR1) or isotype control (ctrl) antibodies. Amount of IFN-γ released is shown as mean±s.d. of triplicate cultures. Results are representative of four independent experiments. (b) THP-1 cells either not infected (no Inf) or infected with the indicated bacteria were used to stimulate three Vα7.2-Jα12 and two Vα7.2-Jα33 MAIT clones. Points represent the amount of IFN-γ released from the indicated T-cell clones and are presented as mean±s.d. Results are representative of three independent experiments. (c) Number of sequences in which theVα7.2gene was found rearranged with individual Jα gene segments. Data were generated by deep mRNA sequencing of lymphocyte-enriched populations from 17 donors. Each point represents a single donor. (d) Vα7.2-Jα12 and Vα7.2-Jα33 MAIT cell clones induced apoptosis inE. coli-infected (E. coli) and not infected (no Inf) THP-1 cells. Infected and not infected THP-1 cells were cultured in the absence of T cells (no T cells) as a control. After 24 h, cells were stained with propidium iodide (PI) and Annexin V, and analysed by flow cytometry after gating for CD3−cells. Numbers indicate the percentage of cells in each quadrant. Results are representative of three independent experiments. (e) Expression of surface CD107a and CD3, and intracellular Granzyme B in two MAIT clones upon co-culture with not infected (grey histogram) orE. coli-infected (white histogram) THP-1 cells. T cells were also cultured in the absence of THP-1 cells (dotted histogram). Results are representative of three independent experiments. (f) Vα7.2-Jα12 and Vα7.2-Jα33 MAIT clones, and a CD1b-restricted T-cell clone specific for a mycobacterial lipid antigen (CD1b-restr.) kill intracellular BCG (left panel) and release IFN-γ (middle panel) and granulocyte macrophage colony-stimulating factor (GM-CSF; right panel). Results are shown as mean±s.d. of triplicate cultures. Colony-forming unit counts and cytokine release were compared with no T-cell group using unpaired Student’st-test. **P≤0.001, ***P≤0.0001. TCRα sequence analysis showed that they all transcribed a functional Vα7.2-Jα12 ( TRAV1-2–TRAJ12 ) rearrangement with identical germline-encoded CDR3 sequence ( Supplementary Table 3 ). Importantly, the same TCRα sequence was found also in three T-cell clones derived from sorted Vα7.2 + CD161 high MAIT cells from a third donor (C) ( Supplementary Table 3 ). We were intrigued by the isolation of such T-cell clones from two different donors; therefore, we investigated the reactivity and the restriction of those T cells. All T-cell clones tested were efficiently stimulated by E. coli -infected THP-1 cells and were restricted by MR1, as anti-MR1-mAbs inhibited their activation ( Fig. 3a ). They were also stimulated by infected Daudi cells, which are naturally β2-microglobulin deficient, following transfection with an MR1-β2m fusion gene construct ( Supplementary Fig. 5 ). Infected wild-type Daudi cells lacking MR1 ( Supplementary Fig. 5a ) did not stimulate Vα7.2-Jα12 or Vα7.2-Jα33 T clones ( Supplementary Fig. 5b ). All T-cell clones expressing the Vα7.2-Jα12 invariant rearrangement also reacted to APC infected with S. aureus and M. smegmatis , which both produce riboflavin precursors [15] , but not to APC infected with Listeria monocytogenes , which does not synthesize riboflavin ( Fig. 3b ). In light of the MR1 restriction and the antigen-responsiveness pattern, we assigned the identified T-cell clones to a new sub-population of semi-invariant MAIT cells. Figure 3: Vα7.2-Jα12 T cells represent a subset of MAIT cells. ( a ) Seven Vα7.2-Jα12 T-cell clones were cultured with THP-1 cells that were either not infected (no Inf), or infected with E. coli in the presence of anti-MR1 (α-MR1) or isotype control (ctrl) antibodies. Amount of IFN-γ released is shown as mean±s.d. of triplicate cultures. Results are representative of four independent experiments. ( b ) THP-1 cells either not infected (no Inf) or infected with the indicated bacteria were used to stimulate three Vα7.2-Jα12 and two Vα7.2-Jα33 MAIT clones. Points represent the amount of IFN-γ released from the indicated T-cell clones and are presented as mean±s.d. Results are representative of three independent experiments. ( c ) Number of sequences in which the Vα7.2 gene was found rearranged with individual Jα gene segments. Data were generated by deep mRNA sequencing of lymphocyte-enriched populations from 17 donors. Each point represents a single donor. ( d ) Vα7.2-Jα12 and Vα7.2-Jα33 MAIT cell clones induced apoptosis in E. coli -infected ( E. coli ) and not infected (no Inf) THP-1 cells. Infected and not infected THP-1 cells were cultured in the absence of T cells (no T cells) as a control. After 24 h, cells were stained with propidium iodide (PI) and Annexin V, and analysed by flow cytometry after gating for CD3 − cells. Numbers indicate the percentage of cells in each quadrant. Results are representative of three independent experiments. ( e ) Expression of surface CD107a and CD3, and intracellular Granzyme B in two MAIT clones upon co-culture with not infected (grey histogram) or E. coli -infected (white histogram) THP-1 cells. T cells were also cultured in the absence of THP-1 cells (dotted histogram). Results are representative of three independent experiments. ( f ) Vα7.2-Jα12 and Vα7.2-Jα33 MAIT clones, and a CD1b-restricted T-cell clone specific for a mycobacterial lipid antigen (CD1b-restr.) kill intracellular BCG (left panel) and release IFN-γ (middle panel) and granulocyte macrophage colony-stimulating factor (GM-CSF; right panel). Results are shown as mean±s.d. of triplicate cultures. Colony-forming unit counts and cytokine release were compared with no T-cell group using unpaired Student’s t -test. ** P ≤0.001, *** P ≤0.0001. Full size image To address whether this novel subset was shared among different individuals, we exploited deep sequencing of total mRNAs to measure the frequency of Vα7.2-Jα12 transcripts within circulating lymphocytes across 17 normal individuals. Total extracted mRNA was used without amplification with TCR-specific primers. In-frame sequences spanning the Vα7.2-Jα region were selected. As these sequences were randomly obtained without previous PCR amplification of mRNA with TCR-specific primers and because of the short reads provided by this method, the number of in-frame sequences recorded was low. Nevertheless, they were deemed sufficient to provide unbiased qualitative and quantitative information about the relative abundance of each different Vα7.2-Jα rearrangement in individual donors. The Vα7.2-Jα33 rearrangements were the most frequent (total of 68 sequences found in 15 out of 17 donors) ( Fig. 3c and Table 3 ) with the predominant amino acid CAVXDSNYQL motif at the V–J junction as previously reported [1] and as found in our Vα7.2-Jα33 MAIT cell clones ( Supplementary Table 3 ). The second most frequent rearrangement was the Vα7.2-Jα12 (total of 37 sequences detected in 8 out of 17 donors) ( Fig. 3c and Table 3 ). All but 1 of the 37 Vα chains possessed an amino acid sequence at V–J junctional regions with the CAVXDSSYKL motif ( Table 3 ) in agreement with that observed also in the Vα7.2-Jα12 T-cell clones ( Supplementary Table 3 ). In some instances, N nucleotides were present together with variable trimming of the Vα and Jα gene segments, resembling the previously reported joining regions in human Vα7.2-Jα33 MAIT cells [1] . A third frequent population was characterized by the Vα7.2-Jα20 rearrangement (12 sequences detected), and in all these V–J junctions an extensive remodelling of germline nucleotides was present, resulting in major junction variability ( Table 3 ). The rearrangements involving other Jα genes were much less frequently represented ( Table 3 ). As a control, the sequences containing the Vα24 gene revealed an expectedly high frequency of the invariant Vα24-Jα18 rearrangement canonical for iNKT cells, thus illustrating the appropriateness of this type of analysis. Therefore, among the T cells expressing the Vα7.2 TCRα chain, together with Vα7.2-Jα33, other populations of T cells expressing a Vα7.2-Jα12 or a Vα7.2-Jα20 rearrangement are significantly represented in the circulating blood of healthy individuals. Table 3 Sequences of V α 7.2-J α 12 ( TRAV1-2-TRAJ12 ) and V α 7.2-J α 20 ( TRAV1-2-TRAJ20 ) rearrangements obtained by RNA deep-sequencing analysis in different donors. Full size table Altogether, these data suggested that T cells with invariant Vα7.2-Jα12 TCR chain represent a second population of human MAIT cells with an apparently similar antigen-responsiveness profile to that described for Vα7.2-Jα33-expressing cells [5] , [6] , [15] , [21] . 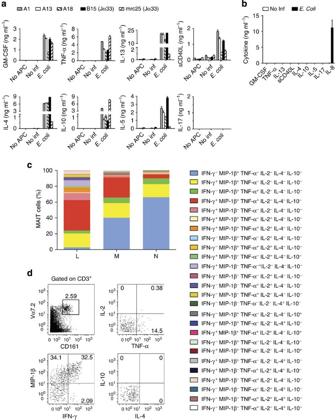Figure 4: Cytokine profile of Vα7.2-Jα12 and Vα7.2-Jα33 MAIT clones, and ofex vivo-stimulated MAIT cells. (a) Multiplex cytokine analysis of Vα7.2-Jα12 and Vα7.2-Jα33 MAIT clones upon co-culture with THP-1 cells either not infected (no Inf) or infected withE. coli(E. coli). Background release of cytokines by unstimulated T cells is also shown (no APC). Data are presented as mean±s.d. of duplicate cultures. (b) Cytokine release profile of not infected andE. coli-infected THP-1 cells in the absence of T cells. THP-1 cells did not release any of the measured cytokines except IL-8, which represented a control of the infection. Data are expressed as mean±s.d. of duplicate cultures. (c) Summary of mass cytometry analysis of MAIT cell functional capacity. Cumulative frequencies of the most common cytokine combinations produced by stimulated cells are coded by colour for each of the three normal donors (L, M, N) tested. (d) Dot plots illustrating the mass cytometry analysis in a representative donor. MAIT cells were gated on CD3+, Vα7.2+and CD161high, and analysed for intracellular expression of the indicated cytokines. Vα7.2-Jα12 MAIT cells are oligoclonal Analysis of the TCRβ amino acid sequences of the six Vα7.2-Jα12 clones revealed that they all expressed gene segments of the Vβ13 (TRBV6) family ( Table 4 ). Furthermore, they were represented by only two different CDR3β clonotypes, which were expressed in four and two clones, respectively ( Table 4 ). These observations suggested that Vα7.2-Jα12 MAIT cells might be biased in their Vβ usage and characterized by a restricted TCRβ repertoire, as for Vα7.2-Jα33 MAIT lymphocytes. To investigate this hypothesis, we determined the frequency of these two CDR3β clonotypes in the cell population from which the clones were generated, taking advantage of the mRNA deep sequencing performed on the same population. Both clonotypes were highly frequent in the Vα7.2 + CD161 high subset, representing 12 and 0.28%, respectively, of the total TCRβ repertoire ( Supplementary Table 2 ). In contrast, these same clonotypes were very rare in the three control non-MAIT populations from the same individual ( Supplementary Table 2 ). These data suggested that the circulating Vα7.2-Jα12 + MAIT cell population is not a rare population in human blood, and moreover is comprises a relatively small number of clonotypes. Table 4 Phenotype and amino acid TCR β sequences of V α 7.2-J α 12 T-cell clones from donor 2B. Full size table Effector functions of Vα7.2-Jα12 + and Vα7.2-Jα33 + MAIT cells To compare the effector functions of Vα7.2-Jα12 and Vα7.2-Jα33 MAIT cell populations, their ability to kill bacterial-infected cells was first assessed. Both MAIT cell types efficiently induced apoptosis in E. coli -infected THP-1 cells ( Fig. 3d ). Importantly, they also induced killing of intracellular mycobacteria and released interferon-γ (IFN-γ) and granulocyte macrophage colony-stimulating factor ( Fig. 3f ), illustrating their capacity for a protective function. This observation was supported by the detection of surface CD107a on T cells, indicating the release of cytotoxic granules, and by the upregulation of intracellular granzyme B expression ( Fig. 3e ). Downregulation of surface CD3 was also observed, consistent with TCR engagement following recognition of infected APC ( Fig. 3e ). We next evaluated the profile of cytokine released by three Vα7.2-Jα12 and two Vα7.2-Jα33 cell clones upon stimulation with E. coli -infected THP-1 cells. Both cell types released Th-0 (granulocyte macrophage colony-stimulating factor), Th-1 (IFN-γ and tumour necrosis factor-α (TNF-α)) and Th-2 (interleukin (IL)-4, IL-5, IL-10 and IL-13)-associated cytokines in an antigen-dependent manner, with no major differences in the profile of cytokines produced between the two groups ( Fig. 4a ). None of the clones released IL-17, while all of them produced soluble CD40L (sCD40L) ( Fig. 4a ). Importantly, the above cytokines were undetectable in the supernatants of E. coli -infected THP-1 cells cultured in absence of T cells ( Fig. 4b ), thus ruling out a possible release by APC. These data suggested that circulating Vα7.2-Jα33 and Vα7.2-Jα12 MAIT cells might contribute to both Th-1 and Th-2 immune responses in peripheral tissues, demonstrating their potential plasticity and immune-regulatory capacity. Figure 4: Cytokine profile of Vα7.2-Jα12 and Vα7.2-Jα33 MAIT clones, and of ex vivo -stimulated MAIT cells. ( a ) Multiplex cytokine analysis of Vα7.2-Jα12 and Vα7.2-Jα33 MAIT clones upon co-culture with THP-1 cells either not infected (no Inf) or infected with E. coli ( E. coli ). Background release of cytokines by unstimulated T cells is also shown (no APC). Data are presented as mean±s.d. of duplicate cultures. ( b ) Cytokine release profile of not infected and E. coli -infected THP-1 cells in the absence of T cells. THP-1 cells did not release any of the measured cytokines except IL-8, which represented a control of the infection. Data are expressed as mean±s.d. of duplicate cultures. ( c ) Summary of mass cytometry analysis of MAIT cell functional capacity. Cumulative frequencies of the most common cytokine combinations produced by stimulated cells are coded by colour for each of the three normal donors (L, M, N) tested. ( d ) Dot plots illustrating the mass cytometry analysis in a representative donor. MAIT cells were gated on CD3 + , Vα7.2 + and CD161 high , and analysed for intracellular expression of the indicated cytokines. Full size image The broad array of cytokines released by the T-cell clones suggested that functionally different populations of MAIT cells exist. To test this hypothesis we investigated six intracellular cytokines on MAIT cells ex vivo in multiparametric analysis using mass cytometry [33] , [34] . In the three tested donors, a large fraction of MAIT cells released MIP-1β, IFN-γ, TNF-α and IL-2 ( Fig. 4c,d ), whereas IL-4 + and IL-10 + cells were less frequent. Cells co-expressing MIP-1β and IFN-γ, MIP-1β and TNF-α, or MIP-1β, IFN-γ and TNFα were abundant. Cells expressing only MIP-1β were also abundant in two donors, while cells expressing only IFN-γ or TNF-α were less represented. All other cytokine combinations were less detected. These findings confirmed that circulating MAIT cells (i) release diverse cytokines, (ii) comprise distinct sub-populations characterized by specific cytokine expression patterns and (iii) display variability of functional sub-populations among individuals. Tissue distribution of MAIT cells We next established a semi-quantitative qPCR technique to study the relative abundance of Vα7.2-Jα33 and Vα7.2-Jα12 transcripts in samples from different tissues. Both transcripts were quantified relative to the amount of total TCR Cα mRNA in PBMC and biopsies of tissues including the liver, kidney, gut, lung, lymph nodes, tonsil, prostate and ovary. A strong signal for MAIT TCR Vα transcripts was detected in PBMC and Vα7.2-Jα33 were the predominant MAIT transcripts ( Fig. 5a ). In the samples analysed, the Vα7.2-Jα12 rearrangement was expressed as a variable fraction, ranging between 0.04 and 0.9% of total TCR Cα transcripts ( Fig. 5a ). Both TCRα MAIT cell transcripts were even more abundant in the liver and in the kidney, with Vα7.2-Jα33 cells being the prevalent subset overall ( Fig. 5a ). In both organs the percentage of Vα7.2-Jα12 transcripts was larger than in peripheral blood ( Fig. 5a,d,e ). In one liver and two kidney samples, the Vα7.2-Jα12 were the only transcripts detected ( Fig. 5d,e ), showing that in some instances, or in some individuals, Vα7.2-Jα12 T cells may overcome Vα7.2-Jα33 T cells. A similar pattern was observed in biopsies from intestine, in which the Vα7.2-Jα12 transcript was also more commonly expressed ( Fig. 5b,g ). 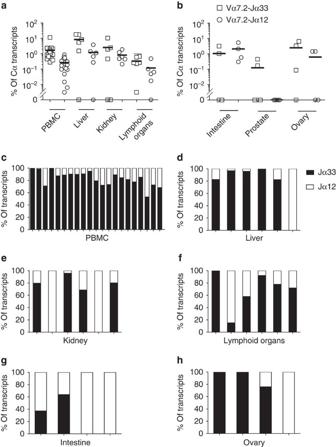Figure 5: Tissue distribution of Vα7.2-Jα33 and Vα7.2-Jα12 cells. (a,b) The percentage of Vα7.2-Jα12 and Vα7.2-Jα33 transcripts among total TCR αβ transcripts in the indicated tissues was assessed by quantitative PCR (qPCR) by quantifying the amount of Vα7.2-Jα12 and Vα7.2-Jα33 amplicons relative to that of TCR Cα amplicon. Horizontal bars indicate the mean value. Relative proportions of Vα7.2-Jα33 and Vα7.2-Jα12 transcripts in (c) PBMC, (d) liver, (e) kidney, (f) lymphoid organs (tonsils, columns 1 and 2, and lymph nodes, columns 3–6), (g) intestine (colon) and (h) ovary. Relative proportions of Vα7.2-Jα12 and Vα7.2-Jα33 transcripts were derived from the qPCR analysis, that is, % of Vα7.2-Jα12 transcripts=% of Vα7.2-Jα12/ (% of Vα7.2-Jα12+Vα7.2-Jα33). Figure 5: Tissue distribution of Vα7.2-Jα33 and Vα7.2-Jα12 cells. ( a , b ) The percentage of Vα7.2-Jα12 and Vα7.2-Jα33 transcripts among total TCR αβ transcripts in the indicated tissues was assessed by quantitative PCR (qPCR) by quantifying the amount of Vα7.2-Jα12 and Vα7.2-Jα33 amplicons relative to that of TCR Cα amplicon. Horizontal bars indicate the mean value. Relative proportions of Vα7.2-Jα33 and Vα7.2-Jα12 transcripts in ( c ) PBMC, ( d ) liver, ( e ) kidney, ( f ) lymphoid organs (tonsils, columns 1 and 2, and lymph nodes, columns 3–6), ( g ) intestine (colon) and ( h ) ovary. Relative proportions of Vα7.2-Jα12 and Vα7.2-Jα33 transcripts were derived from the qPCR analysis, that is, % of Vα7.2-Jα12 transcripts=% of Vα7.2-Jα12/ (% of Vα7.2-Jα12+Vα7.2-Jα33). Full size image Low levels of the two analysed transcripts were detected in lymph nodes and tonsils, where an increase in the relative abundance of Vα7.2-Jα12 transcripts was also noted ( Fig. 5a,f ). In ovary biopsies, the two transcripts were both found ( Fig. 5b ). The Vα7.2-Jα33 and Vα7.2-Jα12 rearrangements were detected in three out of four and two out of four analysed samples, respectively, suggesting differences in the relative proportion of MAIT cells in individual samples ( Fig. 5b,h ). Low levels of Vα7.2 transcripts were present in prostate biopsies, with only the Vα7.2-Jα33 rearrangement detected in two samples out of five individuals ( Fig. 5b ). Biopsies from the lung possessed the fewest TCRαβ cells: in two out of the nine samples in which TCR Cα transcripts were evident, we detected a low level of Vα7.2-Jα33 but not of Vα7.2-Jα12 expression. Altogether, these findings indicated that the two populations of human MAIT cells are abundant in circulating lymphocytes and in a range of tissues, not only the liver and intestine as previously reported [2] , [22] , but also in the kidney and, to a minor extent, lymph nodes, tonsils and ovaries. Vα7.2-Jα12 T cells account for a significant fraction of circulating MAIT cells in adult individuals, and in some donors and/or some tissues they may outnumber classical Vα7.2-Jα33 MAIT cells. The specific influence of polymorphic restriction elements and the variety of stimulatory antigens on the composition of the TCR repertoire remains to be defined. The same issue applies to invariant NKT and MAIT cells, which are restricted to non-polymorphic antigen-presenting molecules and recognize evolutionarily conserved antigens. Oligoclonality is a hallmark of the T-cell populations resident in epithelia and the intestine [23] , [35] , [36] , and a skewed peripheral T-cell repertoire is present in chronic infections [37] , [38] , [39] , autoimmune diseases [40] , [41] and cancer [42] , [43] , [44] . The recent advances in high throughput RNA deep sequencing (RNAseq) technology have enabled investigation of the TCR repertoire in unprecedented detail in both health and disease [45] . Here we applied the RNAseq technique combined with single T-cell cloning to systematically investigate the features of the TCR repertoire of human MAIT cells and in parallel to study their function and antigen responsiveness. We confirmed that the TCRβ repertoire of MAIT cells is strongly skewed towards Vβ2 and Vβ13 chains ( TRBV20 and TRBV6 genes), as suggested by studies performed on small numbers of sequences [1] , [21] . Our study showed a marked oligoclonality of the CDR3β chains in MAIT cells from peripheral blood and normal liver. Unexpectedly, 5% of CDR3β amino acid clonotypes covered on average 80% of the total TCRβ repertoire in MAIT cells; furthermore, ~250 sequences represented 50% of the repertoire, with frequencies of individual clonotypes reaching up to 12% of total MAIT-β sequences. Such frequencies were much higher than those found in non-MAIT control cell populations, which displayed a more heterogeneous Vβ usage and a larger number of unique CDR3β clonotypes. How the extreme oligoclonality of human MAIT cells is generated remains a matter of speculation. The selective expansion of particular clonotypes is probably driven by commensal microbial antigens, as MAIT cells are rare in cord blood, expand early after birth and only then acquire markers of memory T cells [2] , [13] . This possibility is supported by the finding that MAIT cells are not detected in germ-free mice but do appear after colonization of the animal by commensal bacteria [14] . Thus, the oligoclonality of the MAIT cell population might be driven by a combination of non-exclusive factors, probably including a high affinity of the expanded TCR heterodimers for MR1–antigen complexes and the presence of an optimal extracellular stimulatory milieu at the site of antigen recognition. The availability of large numbers of TCR-β sequences allowed a detailed analysis of the individual clonotypes. We did not find amino acid motifs within the CDR3β, although it does contact the MR1-α1 chain [31] , [32] . The absence of conserved motifs is consistent with the known absence of effects on antigen reactivity on single amino acid substitutions in the CDR3β chain of MAIT TCR [30] , [46] . We instead found that MAIT cells displayed a bias in the length of the CD3β domain, with the vast majority of the clonotypes ranging between 11 and 14 amino acids long. This length might be preferentially selected for optimal chain pairing and/or docking on the α1 helix of MR1 (refs 31 , 32 ). The MAIT lymphocyte repertoire was also found to be stable over time, at least across the 5-month interval studied. Thus, the TCR repertoire of MAIT cells is both markedly oligoclonal and stable. A second key finding of our study is the definition of a novel population of MAIT cells expressing an invariant TCR chain and characterized by the Vα7.2-Jα12 rearrangement. These cells shared fundamental traits with ‘conventional’ Vα7.2-Jα33 MAIT cells: (i) they were contained in the MAIT population defined as Vα7.2 + CD161 high , (ii) they were oligoclonal and (iii) they reacted in an MR1-dependent manner only to riboflavin-producing bacteria [15] . Deep RNA sequencing also detected a small number of Vα7.2-Jα20 sequences, previously found to be expressed by rare MAIT cells [10] . These rearrangements were less abundant than Vα7.2-Jα33 and Vα7.2-Jα12, indicative of a third population of MAIT cells. Our data are in agreement with a recent study in which the Vα7.2-Jα12 and Vα7.2-Jα20 chains were found expressed in MAIT cells identified by MR1-tetramer staining [21] . The analysis of the relative abundance of Vα7.2-Jα33 and Vα7.2-Jα12 transcripts within the tissue samples revealed a predominance of the Vα7.2-Jα12 T cells in solid tissues of some individuals, raising the possibility of differences in tissue-homing capacity between the two MAIT cell populations. In some tissues, it appeared that Vα7.2-Jα12 T cells were more abundant than Vα7.2-Jα33 T cells. Whether this differential tissue distribution reflects responsiveness to different types of antigens with unique tissue localization and/or to a different infection history of each donor warrants further investigations. The fact that both MAIT cell populations were present within the kidney and, albeit to a lesser extent, in ovaries, prostate and peripheral lymphoid tissues is interesting in its own right, as these organs are normally sterile in healthy individuals. The question now arises whether MAIT cells accumulate in these tissues following local recognition of microbial antigens, or instead are perhaps autoreactive and recognize antigens specific to these sites. The pattern of cytokines released by Vα7.2-Jα33 and Vα7.2-Jα12 MAIT cell clones in response to E. coli was comparable and was characterized by large amounts of Th0, Th1 and Th2 cytokines, and sCD40L. Both types of MAIT cell efficiently killed E. coli -infected APC and also promoted killing of intracellular mycobacteria. The cytotoxic activity of MAIT cells against infected cells was in accordance with a primary role in controlling pathogen invasion: indeed, in mice infected with Francisella tularensis , MAIT cells accumulate in the lungs and release IFN-γ, TNFα and IL-17A [47] . In addition, their capacity to release regulatory cytokines after bacterial recognition also suggested that MAIT cells might be able to modulate the antimicrobial function of other immune cells, as described for iNKT cells [11] . Perhaps surprisingly, our MAIT cell clones did not release IL-17 in response to bacterially infected APC, reflecting the fact that antigenic stimulation via the TCR is not sufficient to induce a Th-17-like function in these cells [2] , [22] . Instead, activation of this capacity probably requires additional environmental signals, one of which is likely to be IL-7 (ref. 22 ). Multiparametric mass cytometry identified MAIT cell sub-populations co-expressing different cytokines. Most of them produced ex vivo the chemokine MIP-1β (CCL4), which is mostly released by perforin-low memory T cells and facilitates attraction of NK cells, monocytes and other immune cells. Thus, MAIT cells might participate in recruiting other cells to the site of infection and promoting local inflammation. In conclusion, we have shown that MR1-restricted T cells, which use at least two different TCR Vα7.2-Jα chains, exhibit a stable and unexpectedly oligoclonal repertoire in the blood of healthy humans. Their abundance in solid tissues, reactivity to microbial compounds and release of MIP-1β is suggestive of their local protective and immunoregulatory functions. Cells, bacteria and mAbs The following cell lines were used as APC: THP-1, Daudi (both from American Type Culture Collection), Daudi MR1-β2m (described below), monocyte-derived dendritic cell (obtained as described [48] ). APC were infected with either E. coli (DH5α, Invitrogen), S. aureus (MW2, MnCop, LAC, MRSA252, COL), M. smegmatis (mc 2 155, NCTC 8 159) or L. monocytogenes (EGD). The following mAbs specific to human determinants were used for flow cytometry (5 μg ml −1 ): CD4–Pacific blue (PB) (BioLegend) or –fluorescein isothiocyanate (Caltag), CD161–PERCP/Cy5 or –Alexa Fluor 647 (BioLegend, clone HP-3G10), Vα7.2–PE (BioLegend, clone 3C10), CD107a (LAMP-1)–biotin (BioLegend, clone H4A3), CD69–PB (BioLegend, clone FN50), CD3–PB or –PE/Cy7 (BioLegend, clone UCHT1), Granzyme B–fluorescein isothiocyanate (Bio Legend, clone GB11), CD8–PB (Dako) or –PE (BioLegend), AnnexinV–APC (Becton Dickinson), TCRVα24–biotin (C15) TCRVδ2–biotin (4G6), MHC I–unlabelled (W6/32, mIgG2a). Biotinylated mAbs were revealed with streptavidin–PE, –Alexa Fluor 488 or –Brilliant violet 421 (2 μg ml −1 , BioLegend). MR1-specific mAbs 26.5 and 12.2 (both mouse IgG2a) were provided by Ted Hansen, James McCluskey, Marina Cella and Marco Colonna [17] . For flow cytometric experiments, unlabelled mAbs (W6/32, 26.5 and 12.2) were revealed with goat-anti mouse IgG2a–PE (2 μg ml −1 , Southern Biotech). Human samples Human intestine (colon), lung, kidney, ovary, testis, liver, tonsil and lymph node (submandibular and axillary) biopsy samples were obtained from the Pathology Department, University Hospital Basel. The study was approved by the Ethics Committee of Basel (EK: 142/13). Heparinized blood was obtained from healthy donors (age 20–35 years) and PBMC isolated using Ficoll-Paque gradients (Axis-Shield PoC AS). The study was approved by the Ethics Committee of the National University of Singapore (NUS-IRB 09-256 and NUS-IRB 10-250). Liver-associated mononuclear cells were collected from living healthy donors after portal flush using cold preservation solution following removal of the right lobe of donor’s liver. Collection was performed according to the standard protocol preceding liver transplantation [22] . The study was approved by the Ethics Committee of Gleaneagle Hospital, Parkway Health Group, Singapore (PIEC/2012/037). All donors gave written informed consent. Flow cytometry Cell surface labelling was performed according to standard procedures. Intracellular labelling was performed following cell fixation in 2% paraformaldehyde and permeabilization with 0.5% saponin. To measure killing of infected or non-infected APC by T cells, samples were stained with propidium iodide and labelled with anti-CD3 and anti-Annexin mAbs after 24 h of co-culture. For the analysis of CD107a, Granzyme B and CD3 expression, samples were labelled with mAbs specific for these antigens after 4 h of co-culture. Samples were analysed by CyAn ADP flow cytometer (DakoCytomation), with gating to exclude doublets and non-viable cells on the basis of pulse width and incorporation of propidium iodide. Data were analysed using FloJo (TreeStar). Sorting of PBMC and liver T cells from healthy donor samples were carried out using the BD Influx Cell Sorter with BD FACS Software v1.0.0.650 (BD Biosciences). MAIT cell cloning T-cell clones were established from PBMC of normal donors as reported [49] . CD3 + CD4 − Vα24 − Vδ2 − CD161 high cells were sorted from Donor 1 ( Supplementary Fig. 1a ). For other donors, Vα7.2 + CD161 high cells were sorted using anti-Vα7.2 and anti-CD161 mAbs as illustrated in Supplementary Fig. 2 . Sorted cells were cloned by limiting dilution using phytohemagglutinin (l μg ml −1 ) (Wellcome Laboratories), human rIL-2 (100 U ml −1 , Hoffmann-La Roche) and irradiated PBMC (5 × 10 5 ml −1 ). T-cell clones were re-stimulated periodically following the same protocol. Daudi cells expressing MR1A covalently linked with β2m A human MR1A complementary DNA construct linked to β2m via a flexible Gly-Ser linker was generated by PCR using the following primers: Link-MR1-F, 5′-GCGGAGGTGGCAGTGAACGGACGCACTCTCTGAGATATTTTCG-3′; Not I-MR1-cyt-R, 5′-GCGGCCGCTCATCGATCTGGTGTTGGAAGG and Xho I-β2m-F, 5′-CTCGAGATGTCTCGCTCCGTGGCCTTA-3′; Link-β2m-R, 5′-AACCTCCTCCACCCATGTCTCGATCCCACTTA-3′ and Link F, 5′-GAGACATGGGTGGAGGAGGTTCTGGAGGCGGTGGCAGTG-3′; Link R, 5′-GTTCACTGCCACCTCCGCCACTGCCACCGCCTCCAG-3′. The β2m-linker and linker-MR1A were joined together using two-step splicing with overlap extension PCR and the resulting construct subcloned into the Xho I/ Not I sites of the BCMGSNeo expression vector. Daudi cells were transfected by electroporation and selected using G418 (Calbiochem). Killing of intracellular bacteria THP-1 cells were infected with Mycobacterium bovis BCG Pasteur strain (multiplicity of infection=1:5) for 4 h, washed extensively to remove extracellular bacteria and T cells (APC:T cell ratio=1:1) were added. Antibiotic-free medium was used. After 24 h, culture supernatants were harvested for cytokine analysis, and cells were pelleted and lysed with 0.06% SDS for 10 min at room temperature. BCG colony-forming units were counted after 3 weeks by plating serial dilutions on Middlebrook 7H11 agar plates supplemented with 10% oleic-acid-albumin-dextrose-catalase (Difco), in triplicates. Antigen presentation assays APC were incubated with bacteria at a multiplicity of infection of 10 for 3 h at 37 °C in medium without antibiotics, then washed, incubated in medium with kanamycin (100 μg ml −1 ), gentamycin (10 μg ml −1 ) and ciprofloxacin (10 μg ml −1 ) for 1 h, washed again and plated (5 × 10 4 per well). For inhibition assays, anti-MR1 mAbs (26.5) were added (20 μg ml −1 ) to APC after infection and cells were incubated for 1 h before addition of T cells (10 5 per well). Where indicated, APC not infected or infected with E. coli were also cultured in absence of T cells as control. Cytokines released in the supernatants after 24 h were measured by ELISA or by Milliplex Map Kit Human cytokine/chemokine panel I (Millipore). Mass cytometry analysis of cytokine production Cryopreserved human PBMC obtained from three normal donors were thawed and rested overnight before stimulation with phorbol myristate acetate (150 ng ml −1 , Sigma Aldrich) and ionomycin (1 μM, Sigma Aldrich) for 3 h at 37 °C in the presence of brefeldin A (eBioscience) and monensin (BioLegend) to probe for intracellular cytokine production using mass cytometry, performed as previously described using DVS/Fluidigm C5 CyTOF [34] . Surface staining was performed on live cells before fixation, permeabilization with permeabilization buffer (BioLegend) and intracellular cytokine staining. Heavy metal conjugated mAbs specific for the following molecules were used to identify MAIT cells and delineate their functional capacities: CD3 (clone UCHT1, 3 μg ml −1 , Becton Dickinson), Vα7.2 (clone 3C10, 10 μg ml −1 , BioLegend), CD161 (clone HP-3G10, 10 μg ml −1 , BioLegend), IFN-γ (clone 4S.B3, 6 μg ml −1 , BioLegend), MIP-1β (clone D21-1351, 7 μg ml −1 , BD Pharmingen), TNF-α (clone MAb11, 4 μg ml −1 , BioLegend), IL-2 (clone MQ1-17H12, 4 μg ml −1 , BioLegend), IL-4 (clone MP4-25D2, 5 μg ml −1 , BioLegend), IL-10 (clone JES3-12G8, 10 μg ml −1 , eBiosciences). MAIT cell clone TCR sequencing RNA from MAIT cell clones was prepared using the NucleoSpin RNA II Kit (Macherey Nagel) and cDNA synthesized with Superscript III reverse transcriptase (Invitrogen). MAIT cell clone TCRVβ were amplified using a commercial TCRVβ typing amplimer kit (Clontech) as described [50] . MAIT cell clone TCRα were amplified using Vα7.2 (5′-GTCGGTCTAAAGGGTACAGT-3′) and Cα (5′-TTTAGAGTCTCTCAGCTGGTA-3′) primers. PCR-amplified fragments were purified from agarose gel and sequenced. Next-generation sequencing For TCRα and -β high-throughput sequencing, RNA was prepared after TRIzol lysis of sorted cell populations without in vitro culture. Four populations sorted from six donors according to Vα7.2 and CD161 expression were used for TCRβ studies. Total lymphocytes sorted from PBMC of 17 donors were used for TCRα studies. TCRβ analysis: CDR3β regions were amplified and sequenced by Adaptive Biotechnologies Corp. (Seattle, WA) using the ImmunoSEQ assay ( http://www.immunoseq.com ). Briefly, a multiplex PCR system was used to amplify CDR3β sequences from cDNA samples using 52 forward primers for the Vβ gene segment and 13 reverse primers for the Jβ segment. This approach generates a 60-bp fragment capable of identifying the VDJ region spanning each unique CDR3β [51] . Amplicons were sequenced using the Illumina HiSeq platform. Using a baseline developed from a suite of synthetic templates [52] , primer concentrations and computational corrections were used to correct for the primer bias common to multiplex PCR reactions. Raw sequence data were filtered based on the TCRβ V, D and J gene definitions provided by the International Immunogenetics Information (IMGT, www.imgt.org ) database and binned using a modified nearest-neighbour algorithm to merging closely related sequences and remove both PCR and sequencing errors. Data were analysed using the ImmunoSEQ analyser toolset. This approach is capable of detecting one cell in 40,000 T cells using the Survey level, or one cell in 200,000 using the Deep level [53] . TCRα analysis: cDNA libraries were prepared from total RNA. ERCC RNA Spike-In Controls (Life Technologies) were added to the reaction according to manufacturer’s recommendations. The fragmented mRNA samples were subjected to cDNA synthesis using Illumina TruSeqTM RNA sample preparation kit using multiplexing indexes. The pooled cDNA libraries were subjected to a indexed PE sequencing run of 2 × 51 cycles on an Illumina HiSeq 2000. Using this strategy, 30 to 40 millions of paired-end reads were produced for each sample. TCR Vα and Jα region annotation was taken from IMGT and converted to HG19 co-ordinates with UCSC liftover ( http://genome.ucsc.edu/cgi-bin/hgLiftOver ). RNAseq fastq paired-end data were first quality checked with fastqc ( http://www.bioinformatics.babraham.ac.uk/projects/fastqc/ ) and then mapped to an ERCC spike in database with Bowtie, using default parameters except max-insert-size set to 500. Picard tools ( http://picard.sourceforge.net/ ) were used to determine the mean mate distance and s.d. for each sample. The data were then mapped to HG19 with TopHat2 ( http://tophat.cbcb.umd.edu , using default parameters except for the mate information, UCSC annotation as a guide ( http://genome.ucsc.edu/cgi-bin/hgTables?hgsid=337339223 ) and allowing novel junctions. The resulting BAM files and the SAM flags within them were then interrogated with SAMtools ( http://samtools.sourceforge.net/ , to find all reads that mapped in a forward direction on any of the TCR V regions, but for which the mate pair was unmapped (under the assumption this mate pair was mapping across the V–J junction). The unmapped sequences from the TopHat2 mapping were then searched by name to find the sequence for these associated unmapped reads. A synthetic reference database was constructed, which consisted of all possible V and J region fusions, and indexed with Bowtie2. Bowtie2 was then run on this database using the associated unmapped reads with relaxed gap opening/extension penalties (command line parameters —rdg 4,1 —rfg 4,1). A custom script was written, which integrated the resulting BAM file and the CIGAR string within it, with the HG19-converted V and J region annotation from IMGT, to produce an alignment file that displayed these reads in the context of the V–J junction. All of this methodology was written within the Pipeline Pilot frame work ( www.accelrys.com ). Real-time PCR for MAIT cell populations Real-time PCR was performed in a 20-μl reaction volume containing 0.5 μM of each primer and 1 μl of cDNA in Power SYBRgreen MasterMix (Applied Biosystems). For each sample, three reactions were run for Vα7.2-Jα33 and Vα7.2-Jα12 TCR rearrangements and the constant region of TCRα. The following running method was used for PCR: initial incubation for 2 min at 50 °C, incubation for 10 min at 95 °C, 40 cycles of 15 s at 95 °C and 1 min at 60 °C. For the MAIT-cell V–J region-specific and total C-alpha reactions, the following primers were used: Vα7.2Jα33_1Fwd, 5′-GTCGGTCTAAAGGGTACA-3′, Vα7.2Jα33_1Rev, 5′-CCAGATTAACTGATAGTTGCTA; Vα7.2Jα12_1Fwd, 5′-AGTCGGTCTAAAGGGTACAGTT-3′, Vα7.2Jα12_1Rev, 5′-GGTCCCACTCCCGAAGAT; Cα_1Fwd, 5′-ACGCCTTCAACAACAGCATTA-3′, Cα_1Rev, 5′-TCAGGAGGAGGATTCGGAAC-3′. Reactions were run on an ABI 7500 real-time PCR System (Applied Biosystems). Numbers of transcripts were calculated according to the standard curve generated using a cloned full-length TCRα gene (Vα7.2-Jα33 and Vα7.2-Jα12). Results for both populations are represented as a percent of total T cells. Statistical analyses For TCRβ sequence analysis, data were analysed with Mann–Whitney U -test and unpaired Student’s t -test with Welch’s correction. For cytokine and colony-forming unit assays, data were analysed with a two-tailed unpaired Student’s t -test with Welch’s correction. For staining assays, data were analysed with Mann–Whitney–Wilcoxon multiple-comparison test. How to cite this article: Lepore, M. et al . Parallel T-cell cloning and deep sequencing of human MAIT cells reveal stable oligoclonal TCRβ repertoire. Nat. Commun. 5:3866 doi: 10.1038/ncomms4866 (2014). Accession codes: TCRβ deep-sequencing data (ImmunoSeEQ) has been deposited in the NCBI Sequence Read Archive under accession code SRP040254 . Deep RNA-sequencing data set has been deposited in the Gene Expression Omnibus repository under accession code GSE56055 .